Conversion of the LIMA1 tumour suppressor into an oncogenic LMO-like protein by API2–MALT1 in MALT lymphoma MALT1 is the only known paracaspase and is a critical mediator of B- and T-cell receptor signalling. The function of the MALT1 gene is subverted by oncogenic chimeric fusions arising from the recurrent t(11;18)(q21;q21) aberration, which is the most frequent translocation in mucosa-associated lymphoid tissue (MALT) lymphoma. API2–MALT1 -positive MALT lymphomas manifest antibiotic resistance and aggressive clinical behaviour with poor clinical outcome. However, the mechanisms underlying API2–MALT1 -induced MALT lymphomagenesis are not fully understood. Here we show that API2–MALT1 induces paracaspase-mediated cleavage of the tumour suppressor protein LIMA1. LIMA1 binding by API2–MALT1 is API2 dependent and proteolytic cleavage is dependent on MALT1 paracaspase activity. Intriguingly, API2–MALT1-mediated proteolysis generates a LIM domain-only (LMO)-containing fragment with oncogenic properties in vitro and in vivo . Importantly, primary MALT lymphomas harbouring the API2–MALT1 fusion uniquely demonstrate LIMA1 cleavage fragments. Our studies reveal a novel paracaspase-mediated oncogenic gain-of-function mechanism in the pathogenesis of MALT lymphoma. The mucosa-associated lymphoid tissue translocation gene 1 ( MALT1 ) gene encodes the only known paracaspase in the human genome [1] , [2] . The MALT1 protein is a scaffold protein as well as a unique paracaspase involved in antigen-induced nuclear factor-kappa B (NF-κB) signalling and promotes lymphocyte proliferation and survival through cleavage of its substrates [3] , [4] , [5] , [6] . Upon antigen stimulation, the B-cell receptor-associated scaffold protein CARD-containing MAGUK protein 1 (CARMA1), also known as caspase recruitment domain-containing protein 11 (CARD11), is activated to recruit B-cell lymphoma/leukemia 10 (BCL10) and MALT1 forming CARMA1-BCL10-MALT1 (CBM) signallosome via two Ig domains at the amino terminus of MALT1 (refs 3 , 7 , 8 , 9 ). The wild-type MALT1 protein has been found to be an arginine-specific protease by peptide library screening [10] and supported by structural data [11] , [12] . In this regard, MALT1 through its paracaspase domain exhibits proteolytic activity by targeting arginine residues of its substrates, tumour necrosis factor alpha-induced protein 3 (TNFAIP3), also referred to as A20 (ref. 4 ), BCL10 (ref. 6 ), v-rel avian reticuloendotheliosis viral oncogene homologue B (RelB) [13] , cylindromatosis (CYLD) [14] and regnase-1 (ref. 15 ). B-cell receptor stimulation by bacterial antigens such as Helicobacter pylori leads to constitutive activation of MALT1 in the CBM signallosomes and cleavage of these substrates. While the full consequence of these cleavage events is not yet understood, each of the known substrates plays a prominent role in regulating NF-κB [16] and JNK [14] signalling. MALT1 -null animals exhibit B- and T-cell functional defects [17] . On the other hand, constitutive expression of MALT1 in murine models produces a disease resembling human MALT lymphoma [18] . Notably, the paracaspase activity of MALT1 has been demonstrated to be essential for proliferation and survival in some human B cell lymphoma (BCL) subtypes [19] , [20] , [21] , [22] . MALT lymphoma is the most common subtype of malignant lymphoma involving extranodal sites [23] . The t(11;18)(q21;q21) is the most frequent recurrent chromosomal translocation present in MALT lymphomas, and this aberration is associated with antibiotic resistance and aggressive clinical behaviour in gastric MALT lymphomas [1] , [24] , [25] , [26] , [27] . The translocation leads to the juxtaposition of apoptosis inhibitor 2 ( API2) (11q21) to MALT lymphoma translocation gene 1 ( MALT1) (18q21) and the creation of a chimeric fusion API2–MALT1 protein in which the N terminus of API2 is fused to the carboxy terminus of MALT1 (refs 23 , 28 , 29 ). The API2 gene, also known as cIAP2 for cellular inhibitor of apoptosis 2, is a member of the inhibitor of apoptosis protein (IAP) E3 ligase family. API2 protein contains three baculovirus IAP repeat (BIR) domains, a ubiquitin-associated (UBA) domain, a caspase recruitment (CARD) domain and a really interesting new gene (RING) finger domain. After binding to BIR domains, the substrates of API2 are degraded through ubiquitin-proteasome pathways [30] . API2 putatively exerts oncogenic activity through substrate degradation to activate NF-κB and inhibit apoptotic signalling [30] , [31] , [32] , [33] . The API2–MALT1 chimeric protein exhibits constitutive paracaspase activity via auto-oligomerization mediated by the API2 moiety that is independent of CBM signallosome formation [5] , [34] . There are four main breakpoints in the MALT1 gene, including exon 3 (9%), 5 (42%), 7 (32%) and 9 (17%) that are translocated onto exon 7 (93%) of the API2 gene to form E7–E3, E7–E5, E7–E7 and E7–E9 API2–MALT1 fusions. The E7–E3 and E7–E5 fusions still retain one or two Ig domains, while the MALT1 moiety of E7–E7 and E7–E9 fusions lack these domains and thus bypass CBM signallosome-mediated signalling. All of the fusion proteins contain three BIR domains from the API2 N terminus juxtaposed to the paracaspase and Ig domain of the MALT1 C terminus [23] and retain the ability to recruit most substrates of API2 including SMAC, HtrA2/Omi and caspases [35] , [36] . However, despite detailed characterization of the structural aberrations underlying subversion of MALT1 protease function, the mechanisms of API2–MALT1 fusion-induced lymphomagenesis are not well understood. The known substrates of API2–MALT1 include A20 (ref. 4 ), NIK [37] and CYLD [14] . Consistent with the observations in API2–MALT1 cleavage of NIK [37] , we hypothesized that given the retention of the BIR domains in the API2–MALT1 fusions the BIR domains of API2 could recruit atypical substrates to the chimeric API2–MALT1 proteins and that these could be cleaved by the C-terminal MALT1 paracaspase to promote MALT lymphomagenesis via hitherto unknown mechanisms. In this study, we employed an unbiased tandem mass spectrometry-based strategy and discovered that the tumour suppressor LIM domain and actin-binding protein 1 (LIMA1), also known as epithelial protein lost in neoplasm (EPLIN), are novel API2–MALT1 interactors. We further show that LIMA1α is a novel paracaspase substrate of API2–MALT1 and that its cleavage disrupts the tumour suppressor function of LIMA1α. Specifically in this regard, API2–MALT1 paracaspase-mediated proteolysis produces a novel fragment with neo-oncogenic properties in B cells. Our studies indicate a role for LIMA1 deregulation in B-cell lymphomagenesis and highlight a previously unappreciated role of proteolysis in the neomorphic conversion of a tumour suppressor to an oncogenic fragment in the pathogenesis of MALT lymphoma. LIMA1 is a novel binding partner of API2–MALT1 To identify novel mechanisms of API2–MALT1-mediated lymphomagenesis, we generated 293T cells stably expressing FLAG-tagged fusions of API2–MALT1, the paracaspase-inactive API2–MALT1C464A mutant and wild-type MALT1 ( Fig. 1a ). We then analysed immunocomplexes associated with the tagged proteins by liquid chromatography–tandem mass spectrometry (LC–MS/MS) to identify interacting partners of API2–MALT1, the paracaspase-inactive API2–MALT1C464A mutant [4] and MALT1. We confirmed the expression of FLAG fusions ( Supplementary Fig. 1a ) and the expected cleavage of the known substrate A20 ( Supplementary Fig. 1b ) [4] , [37] . One-dimensional SDS–polyacrylamide gel electrophoresis (PAGE) analysis revealed that several bands were shared between the API2–MALT1 and API2–MALT1C464A immunocomplexes ( Fig. 1b ). LC–MS/MS analyses of both API2–MALT1 and API2–MALT1C464A complexes demonstrated efficient co-precipitation of known interactors of API2, SMAC and HtrA2/Omi and TRAF2 ( Fig. 1c ). BCL10 failed to be co-precipitated by the fusion proteins that lack both of the N-terminal Ig domains of MALT1, but was co-precipitated by MALT1 ( Supplementary Fig. 1c ). Importantly, we observed additional distinct bands that repeatedly co-precipitated with catalytically active API2–MALT1 that were absent in the immunoprecipitates of API2–MALT1C464A (25 and 50 kDa; Fig. 1b ). LC–MS/MS analysis identified these bands with high-confidence peptide assignments corresponding to LIMA1 in repeated co-precipitation assays ( Fig. 1b,c ; Supplementary Fig. 1d,e ) and with mass spectral counts comparable to Omi ( Fig. 1c ), but not in immunoprecipitates of MALT1 alone ( Supplementary Fig. 1c ). Taken together, these results suggest that LIMA1 interacts with and is a novel candidate substrate of API2–MALT1. 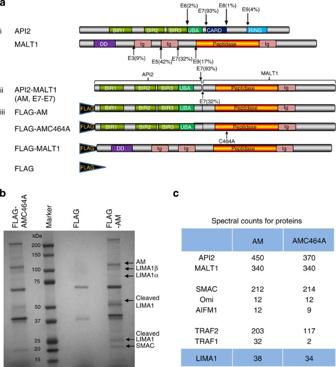Figure 1: Identification of LIMA1 as a novel interactor of API2–MALT1. (a) Schematic diagram of API2, MALT1 and its fusions and FLAG-Wt and mutant. (i) Schematic diagram of API2, MALT1 and fusion breakpoints showing frequency of occurrence. (ii) Schematic diagram of the exon 7–exon 7 fusion. (iii) Schematic diagram of the FLAG-tagged API2–MALT1 (FLAG-AM) and the mutant with the paracaspase-inactivating mutation (FLAG-AMC464A). The functional domains of the proteins are shown as indicated. DD, death domain; E, exon; Ig, immunoglobulin domain; RING, (really interesting new gene) finger domain; UBA, ubiquitin-associated domain. (b) Isolation of API2–MALT1-binding proteins in 293T cells. Cell lysates (20 mg ml−1) were pre-cleared with 50 μl protein A-conjugated beads and mouse IgG1-conjugated beads. The FLAG-API2–MALT1 and FLAG-only immunoprecipitates were resolved on 10% SDS–PAGE and visualized with Coomassie blue staining. (c) Spectral counts of peptides corresponding to LIMA1 and other proteins identified by LC–MS/MS from FLAG-immunopurifications of cells stably expressing FLAG-API2–MALT1 and FLAG-MALT1C464A. Figure 1: Identification of LIMA1 as a novel interactor of API2–MALT1. ( a ) Schematic diagram of API2, MALT1 and its fusions and FLAG-Wt and mutant. (i) Schematic diagram of API2, MALT1 and fusion breakpoints showing frequency of occurrence. (ii) Schematic diagram of the exon 7–exon 7 fusion. (iii) Schematic diagram of the FLAG-tagged API2–MALT1 (FLAG-AM) and the mutant with the paracaspase-inactivating mutation (FLAG-AMC464A). The functional domains of the proteins are shown as indicated. DD, death domain; E, exon; Ig, immunoglobulin domain; RING, (really interesting new gene) finger domain; UBA, ubiquitin-associated domain. ( b ) Isolation of API2–MALT1-binding proteins in 293T cells. Cell lysates (20 mg ml −1 ) were pre-cleared with 50 μl protein A-conjugated beads and mouse IgG1-conjugated beads. The FLAG-API2–MALT1 and FLAG-only immunoprecipitates were resolved on 10% SDS–PAGE and visualized with Coomassie blue staining. ( c ) Spectral counts of peptides corresponding to LIMA1 and other proteins identified by LC–MS/MS from FLAG-immunopurifications of cells stably expressing FLAG-API2–MALT1 and FLAG-MALT1C464A. Full size image Two AKAS motifs mediate LIMA1α binding to the API2 moiety To validate the specific interaction between LIMA1 and API2–MALT1, co-immunoprecipitation and reciprocal immunoprecipitation were performed with anti-FLAG-M2 and anti-V5 beads. Endogenous LIMA1α and LIMA1β both co-precipitated with anti-FLAG in cells expressing FLAG-API2–MALT1 and FLAG-API2–MALT1C464A, but not FLAG alone ( Figs 1c and 2a ). The FLAG-tagged chimeric fusion proteins were reciprocally co-immunoprecipitated by V5-LIMA1α ( Fig. 2b ). V5-LIMA1α co-immunoprecipitated with FLAG-API2–MALT1 and FLAG-API2 (aa1–442), but not with FLAG-MALT1 (full length) and FLAG-MALT1 N-terminal deleted (aa321–824) mutants ( Fig. 2c ). Supplementary Fig. 2a,b shows schematic representations of API2–MALT1, the API2 moiety and the MALT1 moiety. These studies indicate that LIMA1α interacts with API2–MALT1 via the API2 moiety and not with MALT1. LIMA1 contains three known functional domains; a central LIM domain flanked by an actin-binding domain at the N terminus and another actin-binding domain at the C terminus [38] ( Supplementary Fig. 2b ). LIMA1α binds to the API2 moiety of API2–MALT1 via its C terminus since the interaction was abrogated in two C-terminal deletion mutants, but not in the N-terminal actin-binding domain deletion mutant of LIMA1α ( Fig. 2d ). Supplementary Fig. 2b shows a schematic representation of the mutation and deletion mutants. Interestingly, we observed that there are two AKAS motifs (alanine-lysine-alanine-serine, aa350–353 and aa479–482; Supplementary Fig. 2c ) located at the C terminus of LIMA1α. To investigate whether these AKAS motifs represent critical recognition sites in LIMA1α necessary for API2–MALT1 binding, we performed co-immunoprecipitation experiments, which revealed that, compared with LIMA1αWt, the mutants (AKAS1-(A350M), AKAS2-(A479M) and AKAS1-/AKAS2-(A350MA479M) double mutants), in which small alanine residues are substituted with large hydrophobic methionine amino-acid residues [39] , exhibited dramatically reduced binding to API2–MALT1C464A ( Fig. 2e ). From these results, we conclude that the C terminus of LIMA1α contains critical residues for the binding of LIMA1α with the API2 moiety of the API2–MALT1 fusion, and that this interaction is independent of the MALT1 moiety and API2–MALT1 paracaspase activity ( Figs 1c and 2c–f ). 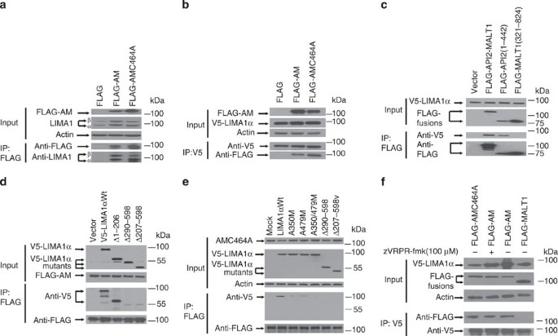Figure 2: Two AKAS motifs mediate LIMA1α binding to the API2 moiety. (a) API2–MALT1 interacts with endogenous LIMA1. Cell lysates (10 mg ml−1) were immunoprecipitated with 25 μl FLAG M2 beads following the same procedures as inFig. 1b. (b) V5-tagged LIMA1α reciprocally co-precipitates FLAG-API2–MALT1. FLAG, FLAG-API2–MALT1 and FLAG-API2–MALT1C464A stably expressing cells were co-transfected with V5-tagged LIMA1α. The chimeric proteins were isolated using V5-conjugated agarose beads and detected with HRP-conjugated anti-FLAG antibody. (c) LIMA1α interacts with the API2 moiety of the API2–MALT1 fusion. LIMA1α, FLAG-API2–MALT1, FLAG-API2 (1–442) and FLAG-MALT1 (321–824) were co-expressed in 293T cells via co-transfection. The V5-LIMA1α-binding activities were demonstrated by co-immunoprecipitation with FLAG-M2 beads (Fig. 1b) and followed with HRP-conjugated anti-V5 immunoblotting. (d) The C terminus of LIMA1α interacts with API2–MALT1. V5-tagged LIMA1αWt and LIMA1α deletion mutants were transfected into cells stably expressing FLAG-API2–MALT1 followed by co-immunoprecipitation and immunoblotting as described inc. (e) The LIMA1α C terminus contains two AKAS motifs that mediate interaction with API2–MALT1C464A. Flag-API2–MALT1C464A and V5-LIMA1αWt and AKAS1 mutation (AKAS1-), AKAS2 mutation (AKAS2-) and double AKAS1 and AKAS2 (AKAS1-2-) mutants were co-expressed in 293T cells. After immunoprecipitation, Flag-API2–MALT1C464A and V5-LIMA1α and its mutants were isolated using anti-Flag-M2 beads and detected by Flag-HRP and V5-HRP, respectively. (f) FLAG-AM and FLAG-AMC464A, but not FLAG-MALT1, were reciprocally co-immunoprecipitated by V5-tagged LIMA1α using anti-V5 agarose beads when co-expressed in 293T cells. Figure 2: Two AKAS motifs mediate LIMA1α binding to the API2 moiety. ( a ) API2–MALT1 interacts with endogenous LIMA1. Cell lysates (10 mg ml −1 ) were immunoprecipitated with 25 μl FLAG M2 beads following the same procedures as in Fig. 1b . ( b ) V5-tagged LIMA1α reciprocally co-precipitates FLAG-API2–MALT1. FLAG, FLAG-API2–MALT1 and FLAG-API2–MALT1C464A stably expressing cells were co-transfected with V5-tagged LIMA1α. The chimeric proteins were isolated using V5-conjugated agarose beads and detected with HRP-conjugated anti-FLAG antibody. ( c ) LIMA1α interacts with the API2 moiety of the API2–MALT1 fusion. LIMA1α, FLAG-API2–MALT1, FLAG-API2 (1–442) and FLAG-MALT1 (321–824) were co-expressed in 293T cells via co-transfection. The V5-LIMA1α-binding activities were demonstrated by co-immunoprecipitation with FLAG-M2 beads ( Fig. 1b ) and followed with HRP-conjugated anti-V5 immunoblotting. ( d ) The C terminus of LIMA1α interacts with API2–MALT1. V5-tagged LIMA1αWt and LIMA1α deletion mutants were transfected into cells stably expressing FLAG-API2–MALT1 followed by co-immunoprecipitation and immunoblotting as described in c . ( e ) The LIMA1α C terminus contains two AKAS motifs that mediate interaction with API2–MALT1C464A. Flag-API2–MALT1C464A and V5-LIMA1αWt and AKAS1 mutation (AKAS1-), AKAS2 mutation (AKAS2-) and double AKAS1 and AKAS2 (AKAS1-2-) mutants were co-expressed in 293T cells. After immunoprecipitation, Flag-API2–MALT1C464A and V5-LIMA1α and its mutants were isolated using anti-Flag-M2 beads and detected by Flag-HRP and V5-HRP, respectively. ( f ) FLAG-AM and FLAG-AMC464A, but not FLAG-MALT1, were reciprocally co-immunoprecipitated by V5-tagged LIMA1α using anti-V5 agarose beads when co-expressed in 293T cells. Full size image API2–MALT1 cleaves LIMA1α to generate a LIM domain-only-like fragment The MALT1 moiety of API2–MALT1 contains the paracaspase catalytic domain that mediates enzymatic cleavage of substrates at arginine residues following a serine residue (SR) [4] , [6] . There are numerous SR and serine lysine (SK) motifs and post-translational modification sites located both N- and C terminal to the central LIM domain within the LIMA1α protein ( Supplementary Figs 2c and 3a ). To further investigate whether LIMA1α is a cleavage substrate of API2–MALT1, V5-tagged LIMA1 was transfected into 293T cells stably expressing FLAG, FLAG-API2–MALT1 or FLAG-API2–MALT1C464A. These experiments revealed that V5-LIMA1α co-precipitated with API2–MALT1 and API2–MALT1C464A, but was cleaved only in the precipitates with API2–MALT1 ( Fig. 3a ). When progressively increasing doses of API2–MALT1 were transiently expressed in cells stably expressing V5-LIMA1α, cleaved LIMA1α fragments were observed in a dose-responsive manner to the levels of API2–MALT1 ( Fig. 3b ). From these data, we surmised that LIMA1α is a novel substrate of the API2–MALT1 oncogenic paracaspase. 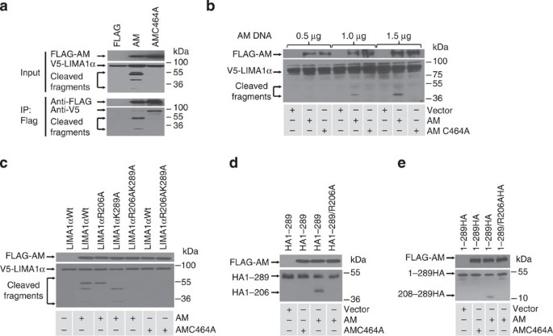Figure 3: API2–MALT1 cleaves LIMA1α at arginine 206 and lysine 289 generating a LMO fragment. (a) Binding and cleavage of V5 N-terminal-tagged LIMA1α when co-expressed with FLAG, FLAG-API2–MALT1 and FLAG-API2–MALT1C464A in 293T cells. The assays with the V5-LIMA1α-transfected cells were carried out as described inFig. 2b. Co-precipitation and cleavage of V5-LIMA1α were detected with HRP-conjugated anti-V5. (b) Dose response of V5-LIMA1α cleavage by API2–MALT1. Cleaved fragments in V5-LIMA1α-expressing cells were detected at 48 h after transfection with 0.5, 1.0 and 1.5 μg API2–MALT1 plasmid DNAs. (c) API2–MALT1 cleaves LIMA1αWt and partially cleaves R206A or K289A single mutants, but not the R206AK289A double mutantin vitro. The catalytically inactive mutant API2–MALT1C464A does not cleave wild-type LIMA1α and API2–MALT1 fails to cleave the LIMA1α R206AK289A double mutant. The synthetic LIMA1αWt and its mutants were incubated with purified API2–MALT1 and API2–MALT1C464A for 2 h at room temperature, and then co-precipitated with FLAG-M2 beads. The co-precipitates were further incubated for 30 min at 30 °C. After elution with 3 × FLAG peptides, the proteolytic cleaved bands were analysed as described in the Methods section. (d) N-terminal HA-tagged LIMA1α aa1–289 was cleaved at R206 when co-expressed with API2–MALT1, but not the R206A mutant, vector control or with the API2–MALT1C464A mutant. The cleaved fragments were detected with anti-HA HRP. (e) The LMO fragment was detected only with anti-HA HRP in cells co-expressing the C-terminal HA-tagged LIMA1α aa1–289 with API2–MALT1, but not in cells co-expressing R206A mutant, nor with vector control or with API2–MALT1C464A. Figure 3: API2–MALT1 cleaves LIMA1α at arginine 206 and lysine 289 generating a LMO fragment. ( a ) Binding and cleavage of V5 N-terminal-tagged LIMA1α when co-expressed with FLAG, FLAG-API2–MALT1 and FLAG-API2–MALT1C464A in 293T cells. The assays with the V5-LIMA1α-transfected cells were carried out as described in Fig. 2b . Co-precipitation and cleavage of V5-LIMA1α were detected with HRP-conjugated anti-V5. ( b ) Dose response of V5-LIMA1α cleavage by API2–MALT1. Cleaved fragments in V5-LIMA1α-expressing cells were detected at 48 h after transfection with 0.5, 1.0 and 1.5 μg API2–MALT1 plasmid DNAs. ( c ) API2–MALT1 cleaves LIMA1αWt and partially cleaves R206A or K289A single mutants, but not the R206AK289A double mutant in vitro . The catalytically inactive mutant API2–MALT1C464A does not cleave wild-type LIMA1α and API2–MALT1 fails to cleave the LIMA1α R206AK289A double mutant. The synthetic LIMA1αWt and its mutants were incubated with purified API2–MALT1 and API2–MALT1C464A for 2 h at room temperature, and then co-precipitated with FLAG-M2 beads. The co-precipitates were further incubated for 30 min at 30 °C. After elution with 3 × FLAG peptides, the proteolytic cleaved bands were analysed as described in the Methods section. ( d ) N-terminal HA-tagged LIMA1α aa1–289 was cleaved at R206 when co-expressed with API2–MALT1, but not the R206A mutant, vector control or with the API2–MALT1C464A mutant. The cleaved fragments were detected with anti-HA HRP. ( e ) The LMO fragment was detected only with anti-HA HRP in cells co-expressing the C-terminal HA-tagged LIMA1α aa1–289 with API2–MALT1, but not in cells co-expressing R206A mutant, nor with vector control or with API2–MALT1C464A. Full size image On the basis of the apparent molecular weights of the LIMA1α fragments observed in cell lysates expressing both API2–MALT1 and LIMA1α ( Fig. 3a,b ; Supplementary Fig. 3b ), we postulated that paracaspase-mediated cleavage may occur at two sites, one within the vicinity of amino-acid residue 200 and the other within the vicinity of amino-acid residue 290. These positions directly flank the LIM domain and both closely neighbour SR/K sites that could represent the precise sites of cleavage (aa206 and 289, respectively). Indeed, when co-expressed with API2–MALT1, R206A substitution in LIMA1α abolished the ~40 kDa cleaved fragment ( Supplementary Fig. 3c ) and K289A substitution prevented formation of the ~50 kDa cleaved fragment ( Supplementary Fig. 3d ). Using an in vitro cleavage assay in a kosmotropic buffer, we observed that LIMA1αWt was only cleaved by purified API2–MALT1, but not API2–MALT1C464A ( Fig. 3c ). While the ~40 kDa and ~50 kDa cleaved fragments were not observed in the cells with R206A and K289A mutations, respectively, the mutant carrying LIMA1αR206AK289A double mutation completely blocked the proteolytic generation of both of these cleaved fragments by purified API2–MALT1 ( Fig. 3c ). API2–MALT1 cleaved LIMA1α at Arg206 and Lys289 generating a LIM domain-only (LMO) fragment evidenced by a band detected at ~10 kDa in API2–MALT1-expressing cells co-transfected with V5-LIMAα1Δ1-206 that still contains the LIM domain at the N terminus ( Supplementary Fig. 3e ). The LMO fragment of LIMA1α generated by specific cleavage is further confirmed by co-expression of API2–MALT1 fusion with LIMA1α (aa1–289) tagged with HA at the N- or C terminus of the protein ( Fig. 3d,e ). The N- or C-terminally tagged deletional mutants aa1–289 are schematically represented in Supplementary Fig. 3f . As expected, the ~40 kDa fragment (aa1–206) and ~10 kDa fragment (aa207–289) were detected only when API2–MALT1 was co-expressed with LIMA1α (aa1–289; Fig. 3d,e ). In the same experiment, expression of the LIMA1α (aa1–289) R206A mutant along with API2–MALT1 abrogated the observed ~40 kDa fragment (aa1–206) and ~10 kDa LMO fragment (aa207–289). Taken together, these observations indicate that API2–MALT1 cleaves LIMA1α at Arg206 and Lys289 with SR/SK motifs ( Supplementary Fig. 3g ) generating a LMO fragment ( Supplementary Fig. 3h ). LIMA1α silencing or cleavage inhibits tumour suppression LIMA1α is a putative tumour suppressor ubiquitously expressed in a variety of tissues and cultured cells ( Supplementary Fig. 4a ) [40] . To investigate LIMA1α protein expression in B cells, we surveyed its expression by western blotting and observed that LIMA1α is expressed in primary human B cells and a broad panel of BCL-derived cell lines ( Fig. 4a ; Supplementary Fig. 4a ). To investigate the biological consequences of functional inactivation of LIMA1α in B cells, we used short hairpin RNA (shRNA) to knockdown the expression of LIMA1 (ref. 41 ). LIMA1 shRNA-mediated stable knockdown resulted in ~90% reduction of LIMA1α expression in L428 B cells and fourfold increase in cell growth ( Fig. 4b-i ). Further, LIMA1α knockdown resulted in a significant increase in colony formation in semi-solid media (approximately twofold; P <0.05, Student’s t -test; Fig. 4b-ii ). LIMA1α depletion also significantly increased fibronectin-mediated L428 cell adhesion (greater than twofold; P <0.01, Student’s t -test; Fig. 4b-iii ) and L1236 cell adhesion (approximately twofold; P <0.05, Student’s t -test; Supplementary Fig. 4b ) and increased L428 B-cell invasiveness (approximately twofold; P <0.05, Student’s t -test; Supplementary Fig. 4c ). These data support a tumour suppressor role of LIMA1α in B cells similar to its known function in epithelial cells [40] , [42] , [43] , [44] . 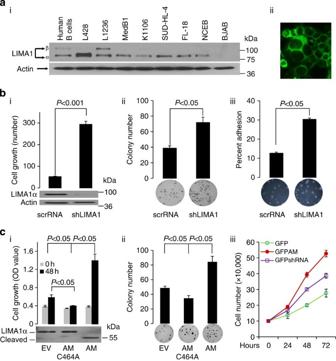Figure 4: Proteolytic cleavage of LIMA1α by API2–MALT1 promotes B-cell lymphomagenesisin vitro. (a-i) Expression of endogenous LIMA1α in non-neoplastic B cells and BCL-derived cell lines. LIMA1 was detected by western blot with rabbit anti-LIMA1 antibody. Actin was used as an internal control. (ii) Distribution of endogenous LIMA1 in L428 B cells stained with rabbit anti-LIMA1 and imaged under microscope ( × 200 magnifications) after staining with Alexa Fluor488 Anti-Rabbit antibody. (b) LIMA1 depletion promotes B-cell proliferation, colony formation and adhesion. (i) LIMA1 knockdown by LentishRNA-mediated silencing increases L428 B-cell proliferation as assessed by WST-1 assay. (ii) L428 cells transduced with LentiscrRNA and LentishRNA against LIMA1 were grown on methylcellulose semi-solid agar for 3 weeks and stained with iodonitrotetrazolium chloride and counted. (iii) L428 cells transduced with LentiscrRNA and LentishRNA against LIMA1 were cultured on fibronectin-coated microtitre plates and attached cells were counted after overnight incubation. (c) API2–MALT1 cleaves LIMA1α to promote B-cell lymphomagenesis. (i) API2–MALT1 cleaves LIMA1α and increases L428 cell proliferation. API2–MALT1 and LIMA1α and/or vector-only constructs were expressed in L428 cells and cell growth was assessed using WST-1 assay. (ii) LIMA1α cleavage is associated with increased colony formation. Cells fromc-ii were used to perform colony formation assays as described inb-ii. (iii) Proliferation of L428 cells expressing API2–MALT1 compared with cells in which LIMA1 is stably depleted using LentishLIMA1. All data are presented as means±s.d. ofn≥3 experimental groups. The valuesP<0.05 andP<0.001 are derived from Student’st-test analysis. Figure 4: Proteolytic cleavage of LIMA1α by API2–MALT1 promotes B-cell lymphomagenesis in vitro . ( a -i) Expression of endogenous LIMA1α in non-neoplastic B cells and BCL-derived cell lines. LIMA1 was detected by western blot with rabbit anti-LIMA1 antibody. Actin was used as an internal control. (ii) Distribution of endogenous LIMA1 in L428 B cells stained with rabbit anti-LIMA1 and imaged under microscope ( × 200 magnifications) after staining with Alexa Fluor488 Anti-Rabbit antibody. ( b ) LIMA1 depletion promotes B-cell proliferation, colony formation and adhesion. (i) LIMA1 knockdown by LentishRNA-mediated silencing increases L428 B-cell proliferation as assessed by WST-1 assay. (ii) L428 cells transduced with LentiscrRNA and LentishRNA against LIMA1 were grown on methylcellulose semi-solid agar for 3 weeks and stained with iodonitrotetrazolium chloride and counted. (iii) L428 cells transduced with LentiscrRNA and LentishRNA against LIMA1 were cultured on fibronectin-coated microtitre plates and attached cells were counted after overnight incubation. ( c ) API2–MALT1 cleaves LIMA1α to promote B-cell lymphomagenesis. (i) API2–MALT1 cleaves LIMA1α and increases L428 cell proliferation. API2–MALT1 and LIMA1α and/or vector-only constructs were expressed in L428 cells and cell growth was assessed using WST-1 assay. (ii) LIMA1α cleavage is associated with increased colony formation. Cells from c -ii were used to perform colony formation assays as described in b -ii. (iii) Proliferation of L428 cells expressing API2–MALT1 compared with cells in which LIMA1 is stably depleted using LentishLIMA1. All data are presented as means±s.d. of n ≥3 experimental groups. The values P <0.05 and P <0.001 are derived from Student’s t -test analysis. Full size image Next we demonstrated using two BCL cell lines that cleavage of LIMA1α by API2–MALT1 mimicked the biological effects observed with shRNA-mediated LIMA1α depletion with significantly increased L428 cell proliferation (approximately threefold; P <0.05, Student’s t -test; Fig. 4c-i ) and colony formation (approximately twofold; P <0.05, Student’s t -test; Fig. 4c-ii ). This cleavage also significantly increased both L1236 cell fibronectin-mediated adhesion ( P <0.05, Student’s t -test) and colony formation ( P <0.05, Student’s t -test; Supplementary Fig. 4d-i, -ii, -iii ). Overexpression of API2–MALT1C464A slightly decreased L428 cell proliferation and colony formation, which may be due to the dominant negative effect that inhibits the endogenous activity of MALT1 in B lymphoma cells [20] , [45] . Interestingly, we observed that L428 cells expressing API2–MALT1 proliferated much faster than the LIMA1α-depleted L428 cells ( Fig. 4c-iii ). We hypothesized that this is due to an autonomous growth-promoting activity intrinsic to the LMO fragment generated by API2–MALT1-mediated cleavage of LIMA1α ( Fig. 3e ; Supplementary Fig. 3f–i ). API2–MALT1 cleavage of LIMA1α yields an LMO-like oncoprotein Comparative sequence analysis revealed that the LMO fragment exhibits 21–29% sequence identity to the N-terminal LIM domain of oncogenic LMO family proteins ( Supplementary Fig. 5a ). Indeed, LMO oncogenes are recurrently targeted by genomic alterations such as translocations and copy number gains [46] , [47] , [48] , [49] , [50] , [51] , [52] , [53] resulting in inappropriate expression of the LMO oncoproteins, and associated with tumorigenesis [54] , [55] , [56] . To investigate the biological effects of the LMO fragment generated by API2–MALT1 in B cells, we expressed the LMO fragment in two different B-cell contexts. We observed that expression of the LMO fragment increased cell proliferation, colony formation and fibronectin-mediated adhesion in L428 B cells ( Fig. 5a-i ). As observed in human primary B cells ( Fig. 4a-i ), primary mouse splenic B cells also express LIMA1 that contains a LIM domain sharing 91.6% sequence identity of the LMO ( Supplementary Fig. 5b,c ). To further establish the oncogenic activity of the LMO-like protein generated by API2–MALT1 cleavage, we directly introduced HA-tagged LMO into freshly isolated primary B cells from C57BL/6 mouse spleens (schematized in Fig. 5b-i ; see Supplementary Fig. 5d,e for western blotting data). Remarkably, while the primary B cells transduced with the control vector were predictably unsustainable in culture and died, the lenti-LMO-transduced cells survived, formed cohesive cellular aggregates and divided continuously beyond 3 weeks ( Fig. 5b-ii ). The ability to transform mouse primary B cells is a strong supportive evidence that the LMO-like protein is neo-oncogenic. Taken together, these results suggest that API2–MALT1 promotes B-cell lymphomagenesis by cleaving LIMA1α to abrogate its tumour suppressor function and by generating a novel LMO fragment that exerts its own intrinsic transforming activity. 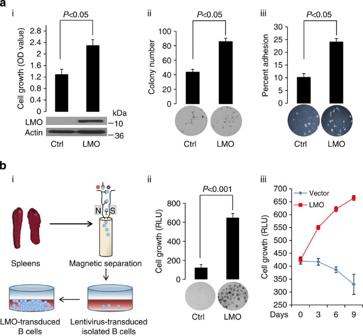Figure 5: LMO of LIMA1α generated by the API2–MALT1 cleavage is an LMO-like oncogenic protein. (a) LMO-like protein promotes B-cell lymphomagenesis. (i) LMO-like protein promotes L428 cell proliferation. L428 cells transduced with LentiGFPLMO and LentiGFP (control) were cultured for 48 h at 37 °C and cell proliferation was determined using the WST-1 assay. (ii) LMO-like protein expression increases colony formation in L428 cells. Stable ectopic expression of LMO was achieved by lentiviral transduction using LentiGFPLMO- and LentiGFP-expressing constructs. Lentivirus-mediated transduction as described in i. (iii) LMO-like protein promotes L428 cell fibronectin-mediated adhesion. Lentivirus-transduced cells are the same as ina-i anda-ii. (b) Primary mouse B-cell transformation by ectopic expression of the LMO-like protein. (i) Schematic of mouse primary B-cell isolation and transduction. LMO-transduced primary mouse B cells show enhanced proliferation. Splenic B cells were isolated using MACS B cell isolation kit and the purity of B cells was determined by immunostaining with FITC-anti-B220. The isolated B cells were transduced with LentiGFPLMO and LentiGFP as described in a-i. Cell viability was determined by CellTiter-Glo Luminescent Cell Viability Assay kit (Promega) every 3 days. (ii) B-cell aggregates reflective of growth were counted by direct visual assessment using light microscope at day 9, and (iii) cell growth was determined using ATP production at days 3, 6 and 9. All data are presented as means±s.d. ofn≥3 experimental groups. The valuesP<0.05 andP<0.001 are derived from Student’st-test analysis. Figure 5: LMO of LIMA1α generated by the API2–MALT1 cleavage is an LMO-like oncogenic protein. ( a ) LMO-like protein promotes B-cell lymphomagenesis. (i) LMO-like protein promotes L428 cell proliferation. L428 cells transduced with LentiGFPLMO and LentiGFP (control) were cultured for 48 h at 37 °C and cell proliferation was determined using the WST-1 assay. (ii) LMO-like protein expression increases colony formation in L428 cells. Stable ectopic expression of LMO was achieved by lentiviral transduction using LentiGFPLMO- and LentiGFP-expressing constructs. Lentivirus-mediated transduction as described in i. (iii) LMO-like protein promotes L428 cell fibronectin-mediated adhesion. Lentivirus-transduced cells are the same as in a -i and a -ii. ( b ) Primary mouse B-cell transformation by ectopic expression of the LMO-like protein. (i) Schematic of mouse primary B-cell isolation and transduction. LMO-transduced primary mouse B cells show enhanced proliferation. Splenic B cells were isolated using MACS B cell isolation kit and the purity of B cells was determined by immunostaining with FITC-anti-B220. The isolated B cells were transduced with LentiGFPLMO and LentiGFP as described in a-i. Cell viability was determined by CellTiter-Glo Luminescent Cell Viability Assay kit (Promega) every 3 days. (ii) B-cell aggregates reflective of growth were counted by direct visual assessment using light microscope at day 9, and (iii) cell growth was determined using ATP production at days 3, 6 and 9. All data are presented as means±s.d. of n ≥3 experimental groups. The values P <0.05 and P <0.001 are derived from Student’s t -test analysis. Full size image Cleavage-resistant LIMA1α suppresses lymphoma growth To further establish the significance of LIMA1α cleavage in API2–MALT1-mediated lymphomagenesis, we reconstituted LIMA1α and its proteolytic-resistant mutant in BJAB B cells in which endogenous LIMA1α is expressed at very low levels ( Fig. 4a-i ). BJAB cells were stably transduced to express API2–MALT1 using an inducible tetracycline-responsive system (BJAB-AM-Tet-On) [37] ( Supplementary Fig. 6a ). In the absence of API2–MALT1 induction, both C-terminal GFP-LIMA1αWt and LIMA1αR206AK289AMut exhibited a predominantly membranous localization when expressed in BJAB-AM-Tet-On cells ( Fig. 6a ) that is consistent with the distribution of endogenous LIMA1 staining in L428 cells ( Fig. 4a-ii ). By contrast, API2–MALT1 induction resulted in a diffuse and predominantly cytoplasmic localization of LIMA1αWtGFP, but did not change the membrane localization of LIMA1αR206AK289AMutGFP ( Fig. 6a ). As expected, API2–MALT1-mediated cleavage reversed the suppressive effects of LIMA1αWt on colony formation (approximately fourfold; P <0.001, Student’s t -test; Fig. 6b-i ). Conversely, API2–MALT1 expression did not reverse the growth suppression or colony formation ( P >0.05, Student’s t -test; Fig. 6b-i ) in the doxycycline-treated LIMA1αR206AK289AMutGFP-transduced BJAB-Tet-On cells. API2–MALT1 is required for the biological transforming effects of LIMA1α cleavage since MALT1 overexpression alone fails to affect the tumour suppression activities of ectopically expressed wild-type LIMA1α in BJAB-Tet-On cells ( Supplementary Fig. 6b,c ). We sought to explore the effects of API2–MALT1 expression on cell cycle progression in the context of LIMA1αWt and LIMA1αR206AK289AMut expression. We found that API2–MALT1 increased the G 2 /M fraction in LIMA1αWt-expressing B cells, but failed to revert LIMA1αR206AK289AMut-induced retardation of cell cycle progression ( Supplementary Fig. 6d–i ). Taken together, these results indicate that API2–MALT1-mediated proteolytic cleavage of LIMA1α contributes to MALT lymphomagenesis. 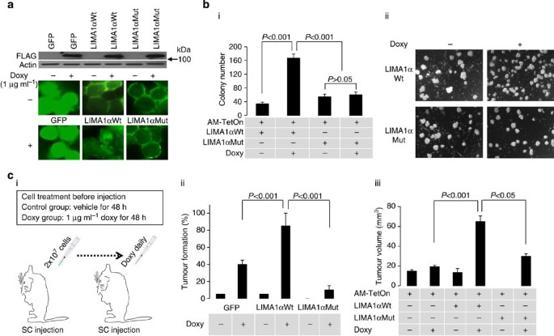Figure 6: Cleavage-resistant LIMA1α suppresses API2–MALT1-induced lymphomagenesis. (a) Doxycycline-induced expression of API2–MALT1 changes the cellular distribution of LIMA1αWtGFP fusion, but not LIMA1αMutR206AK289AGFP fusion. The expression of API2–MALT1 was measured by assessing the intensity of immunoreactive bands yielded from western blotting anti-FLAG after doxycycline induction. The distributions of LIMA1αGFP on cell cytospins were imaged during fluorescence microscopy. (b) Cleavage-resistant LIMA1α mutation impairs colony formation. (i) Colony numbers of LIMA1αWt- and LIMA1αR206AK289AMut-transduced BJAB-AM-Tet-On cells. (ii) Colonies under microscope ( × 200 magnification). Statistical analysis was performed using Student’st-test. Error bars represent ±s.d. (n=3). (c) Paracaspase-resistant LIMA1α mutation impairs BCL growth in xenografted nude mice. Athymic nude mice (n=5 per group) were injected into the flanks with 2 × 107BJAB cells treated with or without doxycycline for 48 h. The injected mice were continuously induced with doxycycline (4 mg per mouse) every 2 days when the tumour formation and growth were observed. (i) Schematic of tumour xenograft in nude mice. (ii) The percentage of mice with tumour formation (the numbers of mice forming tumour/the total numbers of each group × 100%) at day 14 after injection. (iii) The average tumour volume at day 14 after injection into nude mouse xenografts. Statistical analysis was performed using the Studentt-test. Error bars represent ±s.d. (n=10). Figure 6: Cleavage-resistant LIMA1α suppresses API2–MALT1-induced lymphomagenesis. ( a ) Doxycycline-induced expression of API2–MALT1 changes the cellular distribution of LIMA1αWtGFP fusion, but not LIMA1αMutR206AK289AGFP fusion. The expression of API2–MALT1 was measured by assessing the intensity of immunoreactive bands yielded from western blotting anti-FLAG after doxycycline induction. The distributions of LIMA1αGFP on cell cytospins were imaged during fluorescence microscopy. ( b ) Cleavage-resistant LIMA1α mutation impairs colony formation. (i) Colony numbers of LIMA1αWt- and LIMA1αR206AK289AMut-transduced BJAB-AM-Tet-On cells. (ii) Colonies under microscope ( × 200 magnification). Statistical analysis was performed using Student’s t -test. Error bars represent ±s.d. ( n =3). ( c ) Paracaspase-resistant LIMA1α mutation impairs BCL growth in xenografted nude mice. Athymic nude mice ( n =5 per group) were injected into the flanks with 2 × 10 7 BJAB cells treated with or without doxycycline for 48 h. The injected mice were continuously induced with doxycycline (4 mg per mouse) every 2 days when the tumour formation and growth were observed. (i) Schematic of tumour xenograft in nude mice. (ii) The percentage of mice with tumour formation (the numbers of mice forming tumour/the total numbers of each group × 100%) at day 14 after injection. (iii) The average tumour volume at day 14 after injection into nude mouse xenografts. Statistical analysis was performed using the Student t- test. Error bars represent ±s.d. ( n =10). Full size image API2–MALT1 cleaves LIMA1α to promote BCL growth To establish the significance of LIMA1α cleavage in API2–MALT1-mediated lymphomagenesis in vivo , we performed experiments using two different B-cell-derived lines in two different in vivo xenograft models. In this regard, we observed that the proteolytically resistant LIMA1α mutant also retained its tumour suppressive effect in BJAB BCL xenografts in athymic nude mice. In this inducible system, tumour formation and volumes were significantly higher in BJAB-AM-Tet-On cells transduced with LIMA1αWtGFP than in cells transduced with the cleavage-resistant LIMA1αR206AK289AMutGFP under continuous doxycycline induction ( Fig. 6c-i ). To further confirm the consequences of loss of function of LIMA1α and gain-of-function effect of the LMO fragment generated by API2–MALT1 in vivo , we explored the biological effects of API2–MALT1, LIMA1αWt and LIMA1αR206AK289AMut in another xenograft model using L428 cells in SCID-BEIGE mice. In these experiments, L428 cells transduced to express scramble RNA (scrRNA), shLIMA1, API2–MALT1 and LMO, as well as API2–MALT1-LIMA1αWt and API2–MALT1-LIMA1αR206AK289AMut were injected subcutaneously into both dorsal flanks of SCID/BEIGE mice. The volumes of the tumours formed from injected shLIMA1, API2–MALT1, LMO and API2–MALT1-LIMA1αWt-transduced L428 cells were significantly greater than in mice injected with scrRNA or API2–MALT1-LIMA1αR206AK289AMut-transduced L428 cells ( P <0.05, Student’s t -test; Fig. 7a-i ; Supplementary Fig. 7a,b ). These in vivo results using L428 cells in SCID-BEIGE mice corroborate the findings observed using the inducible API2–MALT1 model with BJAB cells xenografted in athymic nude mice, and confirm that API2–MALT1 promotes B-cell lymphomagenesis by cleavage of LIMA1α. 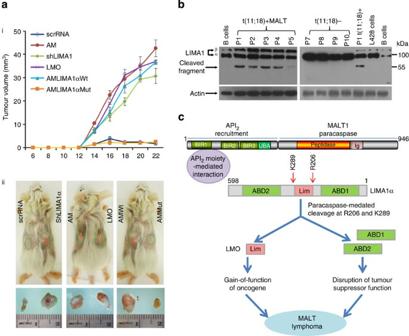Figure 7: API2–MALT1 cleaves LIMA1α to promote B-cell lymphomagenesisin vivo. (a) Cleavage of LIMA1α by API2–MALT1 and cleaved LMO fragment promotes B-cell lymphomagenesisin vivo. Injection of cells into SCID/BEIGE mice and tumour size measurement were performed as described inFig. 6c. (i) Change in tumour volume in L428 cells transduced with recombinant lentiviruses bearing scrRNA, shLIMA1, LMO-like, AM, AM plus LIMA1αWt or LIMA1αR206AK289AMut. The data are presented as means±s.d. ofn=5 experimental groups. (ii) Representative tumours in SCID/BEIGE mice (n=5). (b) Proteolytic cleavage fragments of LIMA1 are present in human MALT lymphomas with t(11;18)(q21;q21) chromosomal aberration, but not in BCLs without the t(11;18)(q21;q21). Evidence of the presence of t(11;18)(q21;q21) in MALT lymphomas was corroborated using a MALT1 break-apart DNA-FISH probe-based strategy (Abbott Molecular; seeSupplementary Fig. 7c). Wild-type (full-length) endogenous LIMA1 and cleavage fragments were detected by western blot with rabbit anti-LIMA1 antibody. Equal quantities of cell lysates (15 μg) from L428 cells and human B cells and patient-derived lymphomas were used in all experiments. (c) Model of API2–MALT1-mediated LIMA1α cleavage and its contribution to B-cell MALT lymphoma pathogenesis. Figure 7: API2–MALT1 cleaves LIMA1α to promote B-cell lymphomagenesis in vivo . ( a ) Cleavage of LIMA1α by API2–MALT1 and cleaved LMO fragment promotes B-cell lymphomagenesis in vivo . Injection of cells into SCID/BEIGE mice and tumour size measurement were performed as described in Fig. 6c . (i) Change in tumour volume in L428 cells transduced with recombinant lentiviruses bearing scrRNA, shLIMA1, LMO-like, AM, AM plus LIMA1αWt or LIMA1αR206AK289AMut. The data are presented as means±s.d. of n =5 experimental groups. (ii) Representative tumours in SCID/BEIGE mice ( n =5). ( b ) Proteolytic cleavage fragments of LIMA1 are present in human MALT lymphomas with t(11;18)(q21;q21) chromosomal aberration, but not in BCLs without the t(11;18)(q21;q21). Evidence of the presence of t(11;18)(q21;q21) in MALT lymphomas was corroborated using a MALT1 break-apart DNA-FISH probe-based strategy (Abbott Molecular; see Supplementary Fig. 7c ). Wild-type (full-length) endogenous LIMA1 and cleavage fragments were detected by western blot with rabbit anti-LIMA1 antibody. Equal quantities of cell lysates (15 μg) from L428 cells and human B cells and patient-derived lymphomas were used in all experiments. ( c ) Model of API2–MALT1-mediated LIMA1α cleavage and its contribution to B-cell MALT lymphoma pathogenesis. Full size image Finally, to demonstrate the clinical relevance of API2–MALT1 targeting LIMA1 in B-cell oncogenesis, LIMA1 proteolytic cleavage was examined by western blot in cell lysates obtained from patient-derived API2–MALT1-positive MALT lymphoma biopsies. As shown in Fig. 7b and Supplementary Fig. 7c , we detected cleaved LIMA1 only in API2–MALT1-positive lymphomas, but not in MALT lymphomas lacking the t(11;18)(q21;q21) chromosomal aberration. Furthermore, ectopic expression of API2-MALT1 in the t(11;18)(q21;q21)-negative marginal zone BCL-derived SSK41 cell line [57] also cleaved LIMA1 and this cleavage was blocked by the paracaspase inhibitor zVRPR-fmk [6] ( Supplementary Fig. 7d ). In parallel, despite abundant expression of endogenous LIMA1α in the MALT1-upregulated but API2–MALT1-negative SSK41 cells, there was no evidence of LIMA1 proteolysis in cells without API2–MALT1 overexpression ( Supplementary Fig. 7d ). Taken together, these results indicate that the API2–MALT1-mediated specific cleavage of LIMA1α and the generation of LMO fragments mechanistically contribute to MALT lymphomagenesis (see Fig. 7c for schematic depiction of the overall findings in this study) ( Supplementary Figs 8–12 contain full scans of western blots displayed in this manuscript). Using a subtractive mass spectrometry-driven proteomic strategy, we discovered that the API2–MALT1 chimeric protein encoded by the t(11;18)(q21;q21) translocation interacts with the LIMA1 tumour suppressor. The recruitment domain of MALT1 at its N terminus replaced by the N terminus of API2 is required for this novel interaction. This interaction is specific since no binding was observed between LIMA1α and MALT1 that interacts with its substrates after formation of the CBM signallosome in response to appropriate stimuli [3] , [7] . We further demonstrated that LIMA1α is proteolytically processed by the paracaspase-mediated activity of API2–MALT1 after binding to the API2 moiety. The API2 moiety in the chimeric fusion recruits LIMA1α via AKAS motifs at its C terminus and MALT1-dependent paracaspase action affects cleavage of LIMA1 resulting in loss of tumour suppressor function. Our studies suggest that API2–MALT1 cleaves LIMA1α at major cleavage site R206 and also at minor cleavage site K289 ( Fig. 3b ). Although unexpected at first, it is plausible that cleavage at K289 by API2–MALT1 may be enhanced by binding of the API2 moiety of the chimeric fusion protein to LIMA1α ( Figs 1b and 3a,c ). Indeed, API2–MALT1 cleavage may occur at additional less preferred sites ( Fig. 3a,c ), but with less catalytic efficiency ( Fig. 3b ). Importantly, we showed that API2–MALT1-induced cleavage disrupts the tumour suppressor function of LIMA1α in vitro ( Figs 4 and 6b ) and in vivo ( Figs 6c and 7a ). Moreover, we observed that API2–MALT1-mediated cleavage of LIMA1α generates an LMO-like protein that demonstrates independent tumorigenic properties in multiple in vitro and in vivo models. While API2–MALT1 cleaves NIK, a regulator of the non-canonical NF-κB signalling pathway [37] , our current demonstration of LIMA1α proteolysis by API2–MALT1 represents the first evidence of a paracaspase-mediated mechanism wherein a wild-type tumour suppressor is cleaved to produce a proteolytic fragment that exhibits its own autonomous oncogenic activity. LIMA1 is a cytoskeleton-associated protein encoded by a gene on band 12q13 and contains a single centrally located lin -11, isl -1 and mec -3 (LIM) domain, flanked by two actin-binding domains each located at the N- and C termini of the wild-type protein [58] . LIMA1 has been recognized as a tumour suppressor based on the multiple mechanisms by which it is targeted for inactivation [40] , [42] , [44] , [59] . LIMA1 protein is preferentially expressed in human epithelial cells and has been observed to be transcriptionally downregulated in epithelial malignancies [40] . Genomic deletions encompassing LIMA1 at the 12q12-13 locus are recurrent in human bronchial and salivary adenoid cystic carcinomas [60] . Further, expression of LIMA1 has been demonstrated to suppress anchorage-independent growth [58] . The biological significance of LIMA1 in cancer is underscored by the fact that loss of expression of LIMA1 in various cancers is correlated with adverse clinical outcomes and inferior survival [37] , [39] , [41] . We demonstrated in two B-cell-derived cell lines that LIMA1α depletion mediated by shRNA promotes cell proliferation, colony formation and ligand-dependent cell adhesion, as did cells ectopically expressing wild-type API2–MALT1, but not those expressing the catalytically defective paracaspase mutant (API2–MALT1C464A). LIMA1α cleavage-dependent tumorigenicity was also diminished in cells co-expressing proteolytically resistant LIMA1α and API2–MALT1 in both in vitro and in vivo xenograft models. The promotion of B-cell oncogenicity observed by API2–MALT1-mediated cleavage of LIMA1α and/or shRNA depletion suggests that LIMA1α functions as a putative tumour suppressor in B cells similar to its known function in epithelial cells. LMO proteins are interacting modules that form multiprotein complexes involved in the regulation of multiple biological processes including erythropoiesis, angiogenesis, cell growth and apoptosis [61] . The LIM domain is a cysteine-rich domain composed of two specialized Zinc fingers that are connected by a two-amino-acid spacer and functions as a modular interface to facilitate protein–protein interactions [62] , [63] , [64] . LMO proteins functioning as candidate oncogenes are known to be recurrently targeted by structural chromosomal alterations including translocations t(11;14)(p15;q11); ( LMO1/-TCR α/δ), t(11;14)(p13;q11);( LMO2-TCR α/δ) and t(7;11)(q35;p13);( LMO2 -TCRβ) occurring in childhood T-cell acute lymphoblastic leukaemias. These translocations are thought to contribute to inappropriate expression of the LMO proteins resulting in leukaemogenesis. The LMO fragment produced by API2–MALT1 exhibits 28% and 26% sequence identities with the N termini of the LIM domains of LMO2 and LMO4, respectively ( Supplementary Fig. 5a ), which are recognized oncogenes known to contribute to the pathogenesis of T-cell leukemia or BCL and breast cancer [65] . This observation is in keeping with our experimental demonstration of the tumorigenic effects of the LMO fragment generated by API2–MALT1-mediated paracaspase cleavage and suggests that this conversion of a growth suppressor into a growth-promoting oncoprotein contributes to API2–MALT1-induced MALT lymphomagenesis. The oncogene-specific nature of this mechanism is supported by our detection of LIMA1 cleavage fragments selectively in t(11;18)(q21;q21) API2–MALT1-expressing patient-derived lymphomas and not in the t(11;18)-negative cases. Our studies highlight novel loss-of-function and gain-of-function mechanisms wherein the normal proteolytic function of a protein is subverted by the juxtaposition of a protein–protein interaction module that recruits unnatural substrates for cleavage, yielding a protein with an independent and opposite biological effect to that of the intact full-length protein from which it was derived. Specifically in this regard, we demonstrate that LIMA1α is a novel interactor and substrate for the API2–MALT1 chimeric paracaspase. While our studies show absence of MALT1 interaction with LIMA1 under basal conditions, it is formally possible that such an interaction may occur after proximal activation and dimerization within the CBM complex. Our findings indicate that in API2–MALT1-expressing lymphomas the API2 moiety of the chimeric fusion recruits LIMA1 and the MALT1 protease domain cleaves LIMA1α. Cleavage of LIMA1α disrupts its tumour suppressor activity and generates a LMO-containing protein that promotes B-cell growth, adhesion and tumorigenicity (schematic model in Fig. 7c ). Overall, these findings suggest that specific inhibition of the interaction between API2 and LIMA1 could lead to the development of targeted therapies for the treatment of API2–MALT1-positive lymphomas. General chemicals and reagents Puromycin (Sigma); doxycycline (Sigma); DNA marker, protein marker, paracaspase inhibitor and protease inhibitors (Roche); arginine (Sigma); protein A/G agarose beads (Santa Cruz); FLAG-M2 beads (Sigma); V5 beads, restriction enzymes and cell culture components RPMI 1640, DMEM, fetal bovine serum (FBS), antibiotics, glutamine, trypsin and FBS were purchased from Invitrogen. Antibodies FLAG conjugated with horseradish peroxidase (HRP; 1:5,000) and rabbit anti-LIMA1 (1:500) were purchased from Sigma. Anti-V5 conjugated with HRP (1:5,000, Invitrogen), anti-HA conjugated with HRP (1:2,000, Thermo Scientific), Donkey HRP-conjugated secondary antibodies against rabbit and mouse as well as FITC-conjugated anti-mouse B220 (1:500, Jackson ImmunoResearch), fluorescence-labelled anti-rabbit and mouse secondary antibodies (1:200, Invitrogen) were used. Plasmids shRNA against LIMA1 (shLIMA1: V2LHS_224834; mature antisense: 5′-AGTGGCTTGGGATGGACAG-3′) and scrRNA were purchased from Open Biosystems. FLAG-API2–MALT1 was inserted into pIRESpuro2 Nhel and NotI cloning sites (University of Cambridge, UK). In the plasmid pIRESGFP bearing FLAG-API2–MALT1, the IRES-controlled puromycin gene was replaced with IRES-controlled green fluorescent protein (GFP). Lentiviral vector pLentiLox RSV was obtained from the viral vector core at the University of Michigan. The packaging plasmids Gagpol, VSVg and Rev were purchased from Invitrogen. Plasmid DNA concentrations were measured using Nanodrop quantitation (Thermo Scientific). Cell culture and establishment of cells stably expressing transduced genes 293T cells (American Type Culture Collection (ATCC)) and 293FT (Invitrogen) were grown in DMEM containing 10% heat-inactivated FBS. BJAB cells (ATCC) were maintained in RPMI 1640 containing 10% heat-inactivated FBS. 293T cells stably expressing FLAG, FLAG-MALT1, FLAG-API2–MALT1 and FLAG-API2–MALT1C464A mutants were developed by the continuous selection with 1 μg ml −1 puromycin (Sigma) after Fugene6 (Roche)-mediated transfection. BJAB-Tet-On cells stably expressing FLAG, FLAG-MALT1 and FLAG-API2–MALT1 were generated at University of Cambridge. The SSK41 cell line was kindly provided by Dr Martin Dyer (University of Leicester, UK). Mouse B cells were isolated with mouse B cell isolation kit (Miltenyi Biotec) by following manufacturer’s protocol and were cultured in RPMI 1640 containing 15% FBS. Plasmid construction and site-directed mutagenesis Human LIMA1α complementary DNA was purchased from Open Biosystems. After amplification by PCR (primers: sense 5′-ATGGAAAATTGTCTAGGAG-3′; antisense 5′-TCACTCTTCATCCTCATCCTC-3′), the forward orientation LIMA1α open reading frame was inserted into pGW8topo vector and then transferred into pcDNA3 N-V5 gateway vector (Invitrogen). V5-LIMA1αΔ1-206 was constructed by generating a BamHI site between R206 and A207 using the GeneTailor Site-Directed Mutagenesis System (Invitrogen) by following the manufacturer’s manual with primer: sense 5′-CAAGCCACTAAGTCCAGATTCGGATCCCTCCAGTCTT-3′; 5′-GAATCTGGACTTAGTGGCTTGGGATGGACAG-3′. V5-LIMA1α aa1–206 and 1–289 were prepared by generating stops after R206 and K289 using site-directed mutagenesis with the primers: 1–206 sense 5′-CACTAAGTCCAGATTCCAGATAGTCCAGTCTT-3′, antisense 5′-TCTGGAATCTGGACTTAGTGGCTTGGGATGGAC-3′; 1–289 sense 5′-CAATCAACTCTTTAAATCTAAGTGAAACTATGATG-3′, antisense 5′-CTTAGATTTAAAGAGTTGATTGAAGTGAGGCTTAC-3′; LIMA1α R206A sense 5′-CAAGCCACTAAGTCCAGATTCCGCAGCCTCCAGTC-3′, antisense 5′-GGAATCTGGACTTAGTGGCTTGGGATGGAC-3′; LIMA1α K289A sense 5′-CTTCAATCAACTCTTTAAATCTGCGGGCAACTATG-3′, antisense 5′-AGATTTAAAGAGTTGATTGAAGTGAGGCTTAC-3′; LIMA1α AKAS1- sense 5′-TCCTGGCTGCAAGTATGGAAATGAAGGCCTCCTC-3′, antisense 5′-TTCCATACTTGCAGCCAGGACACCCACCTTAG-3′; and LIMA1α AKAS2- sense 5′-GAAAGGAAACAGGTGGAAAATATGAAGGCTTCTAAG-3′, antisense 5′-ATTTTCCACCTGTTTCCTTTCTGCAACTCTTCC-3′. LIMA1αR206K289A and LIMA1αAKAS1-AKAS2- multiple mutations were carried out one by one using the primers described above. API2 fragment (1–442): sense 5′-CTGAGGAAAAAGAATCAAATTAGTTATTATTAATC-3′ and antisense 5′-ATTTGATTCTTTTTCCTCAGTTGCTCTTTCTCTC-3′. MALT1 fragment (321–824) was prepared by generating a BamHI site before the fusion point and then all base pairs between this BamHI site and another BamHI site located downstream of FLAG tag at the N terminal of FLAG-MALT1 were removed (University of Cambridge, UK) using primers: sense 5′-GATGAGGCAGTGGAGTGCACTGGATCCGAATTAAATAATC-3′; antisense 5′-AGTGCACTCCACTGCCTCATCTGTTCTTCCTATGATG-3′. The overlapping primers used for the mutations are as follows: API2–MALT1C464A: sense 5′-AATGTGTTCTTATTGGATATGGCTAGGAAAAGAA-3′; antisense 5′-CATATCCAATAAGAACACATTAAGTCCAGTTTC-3′. N-terminal HA-LIMA1α aa1–289 (HA1–289): sense 5′-GGATCCATGTATCCATATGATGTTCCAGATTATGCTGAAAATTGTCTAGGAG-3′; antisense 5′-GCGGCCGCCTACTTAGATTTAAAGAGTTG-3′. The antisense primer for C-terminal HA-LIMA1α aa1–289 (1–289HA): 5′-GCGGCCGCCTAAGCATAATCTGGAACATC ATATGGATACTTAGATTTAAAGAG-3′. HA-LMO: sense 5′-GGATCCATGTATCCATATGATGTTCCAGATTATGCTGCCTCCAGTCTTTCTG-3′. LIMA1αWt, LIMA1αMut, LIMA1α HA1-289 and R206A, LIMA1α 1-289HA and R206A were subcloned into modified pLentiLox RSV at BamHI and NotI sites. LIMA1αWtGFP and LIMA1αMutGFP fusions were created by fused GFP at the C terminal of LIMA1α cloned into BamHI site of the modified pLentiLox RSV. All the PCR fragments and plasmids bearing the mutations were confirmed by DNA sequencing in the DNA Sequencing Core at the University of Michigan. Immunopurification and mass spectrometry analyses Protein lysates from cell lines stably expressing FLAG, FLAG-API2–MALT1 and FLAG-API2–MALT1C464A mutation were prepared with a FLAG-fusion protein purification kit (Sigma) by following the manufacturer’s guidelines. Briefly, cultured cells were harvested, washed three times with ice-cold PBS and resuspended with two volumes of ice-cold Cellytic TMM Cell Lysis Reagent (Sigma, C2978-BULK) containing protease inhibitor cocktail (Roche). After sonication, the protein lysates were obtained by centrifugation at full speed for 30 min at 4 °C and were sequentially filtered with 0.45 μm and then 0.2-μm low-protein-binding filters (Millipore, Millex-HV and Millex-GV). The protein lysates were resuspended at 20 mg ml −1 and pre-precipitated with agarose-conjugated normal mouse IgG1a. In FLAG precipitation assays, FLAG-tagged API2–MALT1 and API2–MALT1C464A added to the protein lysates at 20 mg ml −1 determined by BCA protein assay kit (Thermo Scientific) were immunoprecipitated with 50 μl FLAG-M2 beads after incubation at 4 °C overnight. The FLAG-M2 beads were washed five times with washing buffer (Sigma), then eluted with washing buffer containing 30 μg 3 × FLAG peptides (Sigma) and analysed on SDS–PAGE gel stained with Bio-Safe Coomassie G-250 Stain (Bio-Rad). The binding proteins in the SDS–PAGE were analysed by LC–MS/MS [66] , [67] . Protein expression and in vitro paracaspase cleavage assay V5-tagged LIMA1αWt and LIMA1αMut were synthesized using HeLa cell extracts for high-fidelity cell-free system-coupled transcription, translation, recombinant protein expression and post-translational modification in vitro (Thermo Scientific). Briefly, the BamHI-NotI fragments of LIMA1αWt and mutant DNAs were subcloned into the pT7CFE1 vector. The recombinant LIMA1αWt and mutant were prepared by following the manufacturer’s protocol. In vitro paracaspase cleavage assay was performed as previously described [37] . The purified FLAG-API2–MALT1 fusions from the stably transduced cell lines were co-incubated at 30 °C for 2 h with purified V5-LIMA1α in 50 μl kosmotropic salt buffer (50 mM MES (pH 6.8), 150 mM NaCl, 10% (w/v) sucrose, 0.1% (w/v) CHAPS, 10 mM dithiothreitol and 1 M (NH 4 ) 3 citrate). After incubation at 37 °C for 30 min with constant rotation, an aliquot of the reaction mixture was used for western blotting with a FLAG antibody to verify equal FLAG-API2-MALT1 concentrations. The FLAG-M2 beads were collected, washed with 1 × PBS and boiled for 10 min in 1 × SDS gel loading buffer (with a final concentration of 4% SDS and 300 mM β-mercaptoethanol). Western blotting was performed using the V5 antibody (1:500, sc-58052). Recombinant lentivirus-mediated gene transduction 293T cells were transfected either with Fugene [6] (Roche) or Polyjet (SignaGen Lab) by following the manufacturer’s guidelines. L428 cells were transfected by electroporation. Briefly, 10 5 cells ml −1 were cultured in antibiotic-free RPMI 1640 containing 10% FBS for 48 h. For every single transfection, 10 7 cells were harvested by centrifugation, the pelleted cells were resuspended in 250 μl antibiotic-free RPMI 1640. Before electroporation, the prepared cells were co-incubated for 10 min at room temperature with 50 μl DNA solution (15 μg endotoxin-free DNA in plain RPMI 1640 containing 10 mM HEPES at pH 7.4). The mixture was transferred to a cuvette with a gap of 0.4 cm and electroporated at 230 V and 950 μF with a Bio-rad Gene Pulser (Bio-Rad) [68] . VSVg-pseudotyped recombinant lentivirus production and lentiviral vector-mediated gene transduction Recombinant lentiviruses were produced in 293FT cells (Invitrogen) by following the manufacturer’s protocol. The packaging plasmids Gagpol, VSVg and Rev were purchased from Invitrogen. The resulting recombinant viruses were concentrated by ultracentrifugation at 25,000 r.p.m. (82,700 g ) at 4 °C for 2 h. The titres of the recombinant lentiviruses harbouring reporter GFP were scored by dividing the number of GFP-positive foci at 48 h post-transduction by the dilution factor. The cells were transduced with recombinant lentiviruses at multiplicity of infection of 10 (293T cells) or 50–100 (B cells). The transduced cells carrying GFP reporter were sorted by flow cytometry. Protein concentration determination and immunoblotting The protein concentrations were measured with Pierce BCA Protein Assay Kit (Thermo Scientific, Rockford, IL) by following manufacturer’s guidelines. For western blotting, 10–100 μg proteins were separated on 4–20% Tris-glycine gel running in 1 × MOPS SDS Running Buffer (Novex, Carlsbad, CA). The proteins were transferred overnight at 5 V onto a nitrocellulose membrane (Bio-Rad) using Trans-Blot SD semi-dry transfer cell (Bio-Rad). After 1 h of blocking with 5% milk, the membranes were probed with primary antibodies in 5% milk for 1 h at 37 °C or overnight at 4 °C. The probed membranes were washed five times with PBST (1 × PBS containing 0.1% Tween20) and probed again with HRP-conjugated secondary antibodies. The probed proteins were detected by autography with enhanced chemiluminescence (Thermo Scientific). Immunostaining and fluorescence microscopy The L428 cells and primary mouse B cells were fixed with 4% paraformaldehyde/PBS and permeabilized with 1% Triton 100/PBS for 15 min on ice. After blocking with 5% FBS in PBS containing 1% Triton 100 (PBST buffer), the cells were stained with primary antibodies (1:100) and fluorescently labelled secondary antibodies (1:200). Cell proliferation assays Cell growth curves were generated by directly counting cells or cell aggregates or by using the WST-1 assay (Roche Applied Science, Indianapolis, IN, USA) and/or CellTiter-Glo Luminescent Cell Viability assay (Promega) performed according to the manufacturer’s protocol [69] . Cells were counted using trypan blue exclusion assay. Cell adhesion assay Ninety-six-well plates (Corning) were coated in triplicate with 100 μl freshly prepared fibronectin adhesion-promoting peptides (Sigma, 20 μg ml −1 in ddH 2 O) at 4 °C overnight. Negative control wells were coated with 100 μl BSA (Sigma, 40 μg ml −1 in ddH 2 O). After three washes with PBS containing 0.1% BSA, the plates were blocked with 100 μl RPMI1640 containing 0.5% heat-inactivated FBS for 1 h at 37 °C in a 5% CO 2 incubator. Next, the medium was replaced by 100 μl cell suspensions (10 5 cells ml −1 ) in RPMI160 containing 0.5% heat-inactivated FBS. The unattached cells were removed after 3 h. The attached cells were counted with trypan blue exclusion under a microscope after washing three times with PBS containing 0.1% BSA. Colony formation assay Colony formation assay was carried out in 1% methylcellulose-based media and assessed according to the manufacturer’s protocol (Stemcell Technologies, Vancouver, British Columbia, Canada). After 3 weeks, colonies were stained with iodonitrotetrazolium chloride overnight and counted [69] . Cell transwell migration assay HTS transwell 96-well plates with 5.0 μm polycarbonate membrane (Corning Cat 3388) inserts were coated with rat tail collagen I at 10 μg cm −2 following the manufacturer’s protocol (Sigma). Briefly, the inserts were loaded with 25 μl of diluted collagen solution (0.0572 μg μl −1 ) and air dried in a biological safety cabinet. After removing any remaining collagen solution, the inserts were rinsed once with RPMI1640 containing 0.5% FBS. To set up reservoir wells, 150 μl RPMI1640 containing 10% FBS plus 10 ng stromal cell-derived factor-1α and 0.5% FBS only as negative control were added into each well. Then, 50 μl of 10 5 cells that were serum starved overnight in RPMI1640 containing 0.5% FBS were added to the wells. After overnight incubation at 37 °C and 5% CO 2 , the DAPI (4',6-diamidino-2-phenylindole)-stained GFP-positive cells were counted. In vivo tumorigenicity assay In vivo tumorigenicity was examined in athymic nude and SCID/BEIGE mice [70] . Athymic nude mice (6- to 8-week-old Balb/c nu/nu female) and SCID/BEIGE mice were purchased from the Jackson Laboratory. All animal experiments were done according to a protocol approved by The University Committee on Use and Care of Animals (UCUCA) at the University of Michigan. The mice were injected subcutaneously into both sides of the flanks under ketamine anaesthesia (nude mice: 10 injections per test; SCID/BEIGE mice: 5 injections per test) with 2–5 × 10 7 cells in 0.2 ml mixtures of serum-free RPMI1640 and Matrigel at a ratio of 1:1. Cells were treated with doxycycline (1 μg ml −1 ) for 48 h before injecting into mice. The mice were treated with 4 mg doxycycline every day for 21 days. Tumour formation and growth in the flanks were observed and recorded for 21 days. The tumour sizes of the injected SCID/BEIGE mice were measured every 2 days with a digital caliper (Fowler). The tumour tissues from SCID/BEIGE mice were fixed overnight in 10% neutral buffered formalin, dehydrated in graded concentrations of ethanol and then embedded in paraffin and sectioned. The sections (5-μm thick) were stained with hematoxylin and eosin according to standard protocols and analysed by light microscopy. These tumour sections were imaged under an upright microscope (Olympus BX43). Clinical sample collection and processing API2–MALT1-positive and -negative MALT lymphoma tissues were obtained from the University of Michigan biorepository under a protocol approved by the Institutional Review Board (HUM00023256). Fluorescence in situ hybridization (FISH) was performed as described below. Briefly, nuclei were prepared from paraffin-embedded tissues of API2–MALT1-positive and -negative cases with tissue diagnoses of marginal zone lymphoma. Paraffin-embedded tissue blocks were sectioned at 5 μm, and 3–4 sections were used to prepare nuclei. The sections were deparaffinized twice in xylene for 30 and 10 min, followed by rehydration in 100, 95, 75 and 50% ethanol in water for 5 min each. Tissue sections were digested with Carlsberg solution (0.1% Sigma protease XXIV, 0.1 M Tris, 0.07 M NaCl, pH 7.2) for 1–2 h at 37 °C. The resulting nuclear suspensions were vortexed for 20 min and filtered through a 50-μm nylon mesh. The nuclei were washed once in PBS and fixed in methanol and acetic acid (3:1). For FISH, the nuclear suspensions were pipetted onto Vectabond-treated slides (Vector Laboratories, Burlingame, CA) and air dried overnight. The nuclei were then treated with 50% glycerol/2 3 SSC for 10 min at 90 °C and denatured for 10 min in 70% formamide/2 3 SSC at 70 °C. FISH was performed with the MALT1 DNA-FISH probe purchased from Abbott Molecular according to their protocol. Two hundred or more nuclei were scored from each case. The MALT1 FISH probe generally appears as two distinct signals adjacent to each other (red and green). When there is DNA rearrangement around the API2–MALT1 region, the probe signal splits. FISH was interpreted as normal without rearrangement when two signals without splits were present, aneuploid without rearrangement when more than two signals without splits were present and positive for API2–MALT1 rearrangement when a split signal was present. Statistical analysis All data are presented as mean±s.d. from three or more independent experiments. The statistical significance between two groups was calculated using Student’s t -test. How to cite this article : Nie, Z. et al. Conversion of the LIMA1 tumour suppressor into an oncogenic LMO-like protein by API2–MALT1 in MALT lymphoma. Nat. Commun. 6:5908 doi: 10.1038/ncomms6908 (2015).